Identification of a link between Wnt/β-catenin signalling and the cell fusion pathway Cell fusion has a critical role in various developmental processes, immune response, tissue homeostasis and regeneration, and possibly, in cancer. However, the signals that regulate cell fusion remain poorly understood. In a screen for novel targets of Wnt/β-catenin signalling, we identified glial cells missing 1 ( GCM1 ), which encodes a transcription factor that is involved in epigenetic regulation and is critical for the fusion of syncytiotrophoblast (ST) cells. Here we show that β-catenin/BCL9-Like (BCL9L)/T-cell factor 4 (TCF4) signalling directly targets the GCM1/syncytin pathway and thereby regulates the fusion of human choriocarcinoma cells. Furthermore, we show that the GCM1/syncytin-B pathway is significantly downregulated in the placenta of BCL9L-deficient mice and that the fusion and differentiation of ST-II cells are blocked. Our results demonstrate a signal transduction pathway that regulates cell fusion, and may provide intriguing perspectives into the various biological and pathological processes that involve cell fusion. Cell fusion is an essential and highly regulated event that occurs during development and tissue homeostasis, and is involved in such processes as fertilization, the formation of muscle fibres and bone, development of the placenta in certain species (for example, Primata and Rodentia) and in the development of giant cells in chronic inflammatory reactions [1] , [2] . Furthermore, recent studies have shown that cell fusion has a much broader role in tissue homeostasis and regeneration, such as in the fusion and transdifferentiation of bone marrow-derived cells to neurons, hepatocytes, myocytes and epithelial cells in the intestine [1] , [3] . Advances in the study of cell fusion in tissue repair and regeneration, particularly in inflammatory conditions, have prompted the revival of an earlier theory, which postulates that cell fusion is one of the driving forces of cancer initiation and progression. Cell fusion may facilitate the generation of aneuploidy, multidrug resistance, acquisition of metastatic abilities and provide a source of cancer stem cells [4] , [5] , [6] . Although the molecular mechanisms underlying cell fusion events are not well understood, the most promising candidates for bona fide fusogenic genes in mammals known to date are the syncytin family of genes [2] , [7] , [8] . These are endogenous retroviral genes critical for the fusion of trophoblast cells [9] , [10] , [11] , [12] , [13] . These genes are also suggested to have a role in cell fusion in osteoclast development [7] , cancer development [4] , [5] , [6] and fertilization [14] . Wnt/β-catenin signalling regulates cell fate, proliferation and the self-renewal of stem and progenitor cells, and has critical roles in cancer development [15] , [16] and in the regeneration of various tissues [17] , [18] , [19] , [20] . Canonical Wnt signalling stabilizes β-catenin and induces its association with the T-cell factor (TCF)/lymphoid enhancer factor (LEF) family of transcription factors, thereby activating the transcription of Wnt target genes [15] , [16] . BCL9-Like ( BCL9L , also known as B9L or BCL9-2 ) and BCL9 are vertebrate orthologs of Drosophila legless [21] , [22] , [23] , [24] , an essential component of Wnt/Wingless signalling in flies. Legless functions as an adaptor linking Armadillo ( Drosophila β-catenin) and Pygopus (Pygo), a transcriptional co-activator [21] . However, its precise molecular activities are still controversial [25] . In this study, we show that the β-catenin/BCL9L/TCF4 signalling pathway targets the GCM1/syncytin pathway and thereby regulates cell fusion both in vitro and in vivo . These results demonstrate a signal transduction pathway that links Wnt/β-catenin signalling and cell fusion in mammalian cells for the first time. Identification of GCM1 as a target of β-catenin/TCF complex We searched for novel targets of the β-catenin/TCF complex by chromatin immunoprecipitation (ChIP)-chip (ChIP-combined with high-resolution tiling DNA chip) analysis on SW480 cells, a cell line in which β-catenin/TCF signalling is activated due to a mutated adenomatous polyposis coli gene. We unexpectedly found that β-catenin is associated with a region containing TCF-binding elements (TBEs), 5′-CTTTG(A/T)(A/T)-3′, in intron 2 of the GCM1 gene ( Supplementary Fig. S1 ). GCM1 encodes a transcription factor that is involved in epigenetic regulation through DNA demethylation of CpGs in promoter regions [26] , [27] . This gene transactivates syncytin-1 and -2 and thereby induces cell fusion in trophoblast cells [26] , [28] , [29] , [30] . GCM1 also transactivates Hes5 and induces neural stem cells in the developing brain [27] . However, GCM1 expression was barely detectable in SW480 or in other common cell lines ( Supplementary Fig. S1 ). GCM1 expression is known to be restricted to certain cell types in vivo : for example, in mice, syncytiotrophoblast (ST)-II cells in the placenta, cells in the S3 segment of the proximal tubule of the kidney and certain types of thymic cells [31] , [32] , [33] . Thus, similar to that of syncytin-2 (ref. 26 ), GCM1 expression may be epigenetically silenced by DNA methylation in the promoter region in the majority of the cell types. This assumption is supported by the data from the ENCODE Project [34] showing that CpG sites in the promoter region of GCM1 are methylated in multiple cell lines. It was also shown that the transcription levels of GCM1 in these cell lines are extremely low ( http://genome.ucsc.edu/ENCODE/ ). To investigate whether GCM1 expression is regulated by β-catenin/TCF signalling, we utilized the human trophoblastic choriocarcinoma cell line BeWo, which is known to express GCM1 . This cell line is frequently used as a model system for studying ST-like differentiation and cell fusion induced by treatment with forskolin (FK) [35] , an adenylate cyclase activator. It is known that FK treatment of BeWo cells upregulates the expression and activity of GCM1 (refs 28 , 29 , 36 ). Furthermore, FK treatment or other PKA activators are known to activate the canonical Wnt pathway in multiple cell lines by either stabilizing β-catenin [37] or by promoting β-catenin binding to its co-activator CREB-binding protein [38] . We therefore examined whether FK treatment activates β-catenin/TCF signalling in BeWo cells. Using a reporter plasmid that contains optimal (TOP) or mutant (FOP) TCF-binding sites upstream of a luciferase gene, we found that FK treatment for 48 h significantly activates the TOP reporter compared with the FOP reporter ( Fig. 1a ). This activation was inhibited by small-interfering RNA (siRNA)-mediated knockdown of β-catenin. Furthermore, qRT–PCR analysis revealed that FK treatment upregulated Wnt target genes such as AXIN2 , BAMBI and LEF1 ( Fig. 1b ). In addition, the amounts of β-catenin, BCL9L and the modified active form of TCF4 (refs 39 , 40 ) in the nuclear fraction were increased significantly in response to FK treatment ( Fig. 1c ). These results suggest that β-catenin/BCL9L/TCF signalling is activated in FK-treated BeWo cells. 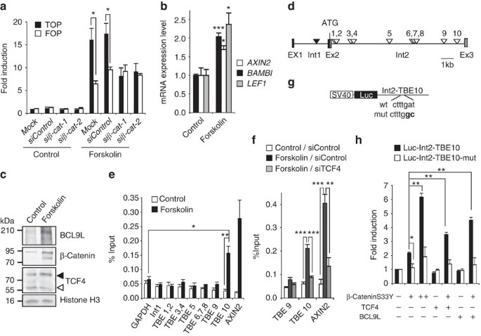Figure 1:GCM1is a direct transcriptional target for β-catenin/BCL9L/TCF4 signalling. (a) BeWo cells transfected with the indicated siRNAs were treated with 50 μM FK or vehicle (control) for 48 h and assayed for TOP or FOP activities. siβ-cat-1, -2 denote siRNAs targeting different sites of β-catenin mRNA. (b) qRT–PCR analysis of the expression levels of Wnt target genes in FK-treated BeWo cells. (c) Portions of nuclear lysates prepared for ChIP assays were analysed by immunoblotting. The closed and open triangles indicate 80 kDa (modified) and 60 kDa TCF4s, respectively. Representative data from three independent experiments are shown. (d) Schematic representation of the genome structure ofGCM1. Open and closed triangles indicate TBEs and a negative control region containing no TBEs within a region 1 kb up- or downstream, respectively. Ex, Exon; Int, Intron. (e,f) ChIP assays with anti-β-catenin antibody.GAPDHandAXIN2are negative and positive controls, respectively. (g) Schematic representation of the luc-Int2-TBE10 and luc-Int2-TBE10-mut reporter constructs for enhancer assays. (h)Cis-activation potential of the region containing TBE10 or its mutant in response to β-catenin/BCL9L/TCF4 signalling was evaluated by luciferase enhancer assays. Values are shown as mean±s.e.m. *P<0.05; **P<0.01; ***P<0.001.N=3 (a,b,e) orN=4 (f,h). Statistical tests were performed using unpaired two-tailed Student'st-test. Figure 1: GCM1 is a direct transcriptional target for β-catenin/BCL9L/TCF4 signalling. ( a ) BeWo cells transfected with the indicated siRNAs were treated with 50 μM FK or vehicle (control) for 48 h and assayed for TOP or FOP activities. siβ-cat-1, -2 denote siRNAs targeting different sites of β-catenin mRNA. ( b ) qRT–PCR analysis of the expression levels of Wnt target genes in FK-treated BeWo cells. ( c ) Portions of nuclear lysates prepared for ChIP assays were analysed by immunoblotting. The closed and open triangles indicate 80 kDa (modified) and 60 kDa TCF4s, respectively. Representative data from three independent experiments are shown. ( d ) Schematic representation of the genome structure of GCM1 . Open and closed triangles indicate TBEs and a negative control region containing no TBEs within a region 1 kb up- or downstream, respectively. Ex, Exon; Int, Intron. ( e , f ) ChIP assays with anti-β-catenin antibody. GAPDH and AXIN2 are negative and positive controls, respectively. ( g ) Schematic representation of the luc-Int2-TBE10 and luc-Int2-TBE10-mut reporter constructs for enhancer assays. ( h ) Cis -activation potential of the region containing TBE10 or its mutant in response to β-catenin/BCL9L/TCF4 signalling was evaluated by luciferase enhancer assays. Values are shown as mean±s.e.m. * P <0.05; ** P <0.01; *** P <0.001. N =3 ( a , b , e ) or N =4 ( f , h ). Statistical tests were performed using unpaired two-tailed Student's t -test. Full size image To confirm the results of the ChIP-chip analysis, we performed ChIP–qPCR analyses on FK-treated BeWo cells using an antibody against β-catenin. Among 10 TBEs within 11.2 kbp of intron 2 of GCM1 ( Fig. 1d ), β-catenin was found to bind to a region containing TBE number 10 (TBE10) in a FK-dependent manner ( Fig. 1e ), consistent with the result from CHIP-chip analysis. In a parallel experiment, β-catenin was also found to bind to the transcription start site in AXIN2 , which contains a TBE ( Fig. 1e ). Furthermore, knockdown of TCF4 resulted in a significant decrease in β-catenin binding to these regions ( Fig. 1f ). We next investigated the cis -activating potential of the region containing TBE10 in enhancer assays by inserting this region downstream of a reporter cassette consisting of the SV40 promoter and luciferase gene ( Fig. 1g ). Co-transfection of this reporter into BeWo cells together with a constitutively active mutant of β-catenin, β-catenin-S33Y, resulted in a significant increase in the reporter activity ( Fig. 1h ). Furthermore, co-expression of either TCF4 or BCL9L along with β-catenin-S33Y resulted in the synergistic enhancement of the reporter activity ( Fig. 1h ). A mutated TBE10 construct showed significantly lower activity in these assays ( Fig. 1g,h ). These results suggest that GCM1 expression is directly regulated by β-catenin/BCL9L/TCF signalling through targeting TBE10 in intron 2 of GCM1 . Interestingly, intron 2 of mouse Gcm1 has been postulated to contain an enhancer region critical for establishment of its expression pattern [41] . Among seven TBEs within intron 2 of mouse Gcm1 , TBE5 and TBE7 are highly and moderately conserved compared with human TBE6 and TBE10, respectively, ( Supplementary Fig. S1 ). In addition, mouse TBE7 and human TBE10 both reside in similar location, ca. 630 bp upstream of the intron 2–exon 3 junction. Thus, mouse TBE7 may correspond to human TBE10. β-catenin signalling regulates FK-induced cell fusion We further investigated whether the endogenous GCM1/syncytin pathway is regulated by β-catenin/BCL9L/TCF signalling. siRNA-mediated knockdown of BCL9L, β-catenin or TCF4 in FK-treated BeWo cells all resulted in a significant downregulation of FK-induced expression of GCM1 , syncytin-1 and syncytin-2 ( Fig. 2 ), as well as AXIN2 ( Supplementary Fig. S2 ). It has been reported that upregulation of GCM1 , syncytin-1 and syncytin-2 are required for FK-induced fusion of BeWo cells [29] , [42] . We therefore examined whether β-catenin/BCL9L/TCF signalling is required for FK-induced fusion of BeWo cells. Knockdown of BCL9L, β-catenin or TCF4 significantly decreased the number of cell fusion events among FK-treated BeWo cells ( Fig. 3 ), but did not inhibit gross morphological changes, such as enlargement of the cells or extension of protrusions. Thus, β-catenin/BCL9L/TCF signalling is required for FK-induced cell fusion but not for morphological changes. Taken together, these results suggest that β-catenin/BCL9L/TCF signalling regulates cell fusion through targeting the GCM1/syncytin pathway. 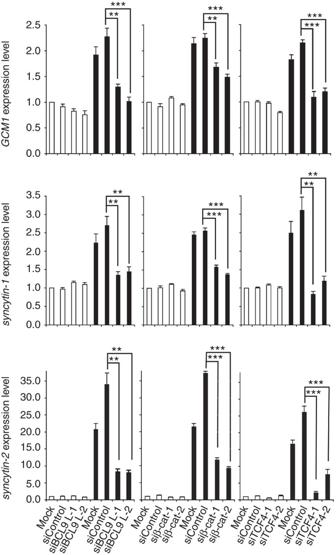Figure 2: β-Catenin/BCL9L/TCF4 signalling targets theGCM1/syncytin pathway in BeWo cells. qRT–PCR analysis of the effect of BCL9L, β-catenin or TCF4 knockdown on FK-inducedGCM1,syncytin-1andsyncytin-2expression. Values were normalized byGAPDHexpression level and are shown as fold increase against mock control. Si (gene symbol) -1 and -2 denote siRNAs targeting different sites of the mRNA. Values are shown as mean±s.e.m. **P<0.01; ***P<0.001.N=4. Statistical tests were performed using unpaired two-tailedt-tests. Open bars, control; closed bars, FK. Figure 2: β-Catenin/BCL9L/TCF4 signalling targets the GCM1 /syncytin pathway in BeWo cells. qRT–PCR analysis of the effect of BCL9L, β-catenin or TCF4 knockdown on FK-induced GCM1 , syncytin-1 and syncytin-2 expression. Values were normalized by GAPDH expression level and are shown as fold increase against mock control. Si (gene symbol) -1 and -2 denote siRNAs targeting different sites of the mRNA. Values are shown as mean±s.e.m. ** P <0.01; *** P <0.001. N =4. Statistical tests were performed using unpaired two-tailed t -tests. Open bars, control; closed bars, FK. 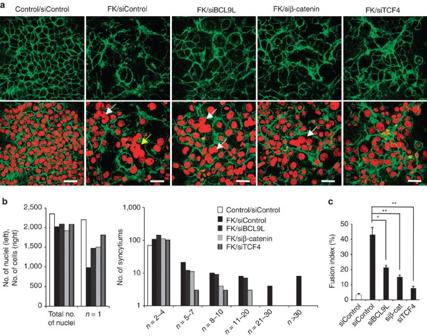Figure 3: β-Catenin/BCL9L/TCF4 signalling is required for FK-induced fusion of BeWo cells. (a) The effect of BCL9L, β-catenin or TCF4 knockdown on the extent of cell-cell fusion of BeWo cells after 48 h of FK treatment was analysed by immunostaining with anti-plakoglobin antibody (green) and TO-PRO-3 nuclear staining (red). Staining of plakoglobin is shown separately in top panels to clarify the inter-cellular boundaries. White arrows, syncytium with >4 nuclei; yellow arrow, syncytium with >10 nuclei. Scale bars, 50 μm. (b) Distribution of syncytia as a function of the number (n) of nuclei per cell or syncytium. The number of nuclei per syncytium were quantified and plotted. In the right panel,y-axis is in a logarithmic scale. (c) Cell-cell fusion events were quantified and shown as fusion indexes. The extent of cell fusion was calculated as a fusion index of [(N−S)/T]×100%, where (N−S) equals the number of fusion events,Nis the number of nuclei in the syncytia,Sis the number of syncytia andTis the total number of nuclei counted. Open bars, control, closed bars FK. Values are shown as mean±s.e.m. *P<0.05; **P<0.01.N=3. Statistical tests were performed using unpaired two-tailed Student'st-test. Full size image Figure 3: β-Catenin/BCL9L/TCF4 signalling is required for FK-induced fusion of BeWo cells. ( a ) The effect of BCL9L, β-catenin or TCF4 knockdown on the extent of cell-cell fusion of BeWo cells after 48 h of FK treatment was analysed by immunostaining with anti-plakoglobin antibody (green) and TO-PRO-3 nuclear staining (red). Staining of plakoglobin is shown separately in top panels to clarify the inter-cellular boundaries. White arrows, syncytium with >4 nuclei; yellow arrow, syncytium with >10 nuclei. Scale bars, 50 μm. ( b ) Distribution of syncytia as a function of the number ( n ) of nuclei per cell or syncytium. The number of nuclei per syncytium were quantified and plotted. In the right panel, y -axis is in a logarithmic scale. ( c ) Cell-cell fusion events were quantified and shown as fusion indexes. The extent of cell fusion was calculated as a fusion index of [( N − S )/ T ]×100%, where ( N − S ) equals the number of fusion events, N is the number of nuclei in the syncytia, S is the number of syncytia and T is the total number of nuclei counted. Open bars, control, closed bars FK. Values are shown as mean±s.e.m. * P <0.05; ** P <0.01. N =3. Statistical tests were performed using unpaired two-tailed Student's t -test. Full size image Characterization of the phenotypes of Bcl9l -deficient mice To investigate the role of Wnt/β-catenin signalling in the regulation of the GCM1/syncytin pathway in vivo , we took advantage of Bcl9l -deficient mice generated by gene targeting ( Supplementary Fig. S3 ). Bcl9l +/− mice were healthy and fertile, whereas Bcl9l −/− mice died at around embryonic day (E) 10.5–11 ( Supplementary Table S1 ). Gross morphology, cardiovascular development, the number of somites and blood flow of Bcl9l −/− concepti at E9.5 appeared normal ( Supplementary Fig. S4 ). However, at E10.5, Bcl9l −/− embryos were smaller than their littermates ( Supplementary Fig. S4 ) and possessed fewer somites (37±1.2 for wild-type; 30±1.5 for Bcl9l −/− ; mean±s.d. ; N =8 for each genotype; P <10 −7 ; unpaired two-tailed Student's t -test), indicating that their growth was arrested at around E10. Furthermore, the placenta and yolk sac became pale in Bcl9l −/− concepti ( Supplementary Fig. S4 ). By E11.5, Bcl9l −/− embryos had become fragile and were resorbed ( Supplementary Fig. S4 ). As most of these phenotypes are similar to those frequently seen in mutant mice with placental defects, we focused our analysis on the placenta. The labyrinth layer functions as a site for the exchange of gases and nutrients between maternal and fetal blood in the placenta [41] , [43] . Bcl9l −/− placenta showed normal morphology at E8.5, and chorioallantoic attachment occurred normally ( Fig. 4 ; Supplementary Fig. S4 ). However, at E9.5 and 10.5, branching morphogenesis of the chorionic plate and subsequent invasion of the fetal blood vessels were virtually abrogated ( Fig. 4a–h ). By contrast, the morphology, growth and distribution of the spongiotrophoblast and trophoblast giant cells appeared normal ( Fig. 4i,j ). These results indicate that the growth arrest and subsequent death of Bcl9l −/− embryos at the mid-gestation are caused by an oxygen and/or nutritional deficit that result from the failure of the functional labyrinth layer to form in the placenta. 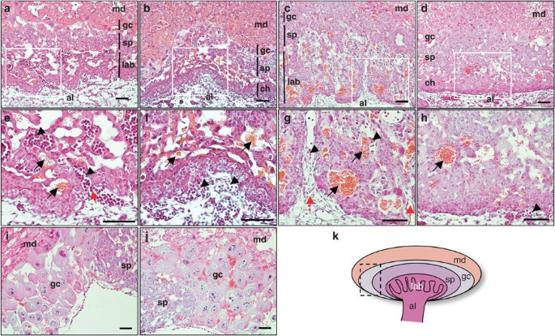Figure 4: Complete block of branching morphogenesis and labyrinth layer formation inBcl9l−/−placenta. (a–j) Haematoxylin and eosin staining of placental sections from E9.5 (a,b) and E10.5 (c,d,i,j) concepti. (a,c,i) Wild-type. (b,d,j)Bcl9l−/−. The boxed areas in panelsa––dare shown at higher magnification in panelse–h, respectively. Panelsa–hshow the central area of the placentas where chorioallantoic attachment occurred. Panelsi,jshow the lateral area of the placentas where trophoblast giant cells are abundant. (k) Schematic representation of the layered structure of the placenta. The dotted box denotes areas shown in (i,j). Arrowheads, nucleated fetal red blood cells; black arrows, maternal red blood cells; red arrows, fetal blood vessels invading chorionic plate. al, allantois; ch, chorionic plate; gc, trophoblast giant cells; lab, labyrinth layer; md, maternal decidua; sp, spongiotrophoblast. Scale bars, (a,b,eandf) 50 μm; (c,dandg–j) 100 μm. Figure 4: Complete block of branching morphogenesis and labyrinth layer formation in Bcl9l−/− placenta. ( a – j ) Haematoxylin and eosin staining of placental sections from E9.5 ( a , b ) and E10.5 ( c , d , i , j ) concepti. ( a , c , i ) Wild-type. ( b , d , j ) Bcl9l −/− . The boxed areas in panels a –– d are shown at higher magnification in panels e – h , respectively. Panels a – h show the central area of the placentas where chorioallantoic attachment occurred. Panels i , j show the lateral area of the placentas where trophoblast giant cells are abundant. ( k ) Schematic representation of the layered structure of the placenta. The dotted box denotes areas shown in ( i , j ). Arrowheads, nucleated fetal red blood cells; black arrows, maternal red blood cells; red arrows, fetal blood vessels invading chorionic plate. al, allantois; ch, chorionic plate; gc, trophoblast giant cells; lab, labyrinth layer; md, maternal decidua; sp, spongiotrophoblast. Scale bars, ( a , b , e and f ) 50 μm; ( c , d and g – j ) 100 μm. Full size image The expression of Gcm1 , syncytin A ( Syna ) and syncytin B ( Synb ) is known to be restricted to specific ST and its precursor cells in the developing placenta [32] , [33] . We therefore examined the spatiotemporal expression pattern of Bcl9l in the placenta by β-galactosidase (β-gal) staining, utilizing the lacZ gene inserted in-frame downstream of the Bcl9l promoter ( Supplementary Fig S3 ). At E8.5 in the chorionic plate, β-gal expression was restricted to the basal cells lining the chorioallantoic interface ( Fig. 5a ), which are postulated to include ST-II precursor cells [33] , [44] . At E9.5, we further observed staining of the elongated differentiating ST-II cells at the innermost layer of the invagination ( Fig. 5b,c ; Supplementary Fig. S5 ), and at E10.5, staining of the thin layer of ST surrounding the fetal capillaries ( Fig. 5d,e ). By contrast, β-gal staining of Bcl9l −/− placentas at E10.5 revealed that cells having Bcl9l promoter activity remained lined at the basal chorionic plate and did not go through morphological changes seen in Bcl9l +/− placentas ( Fig. 5f ). Throughout the stages examined, low to moderate levels of β-gal expression were also observed in the allantoic mesoderm. 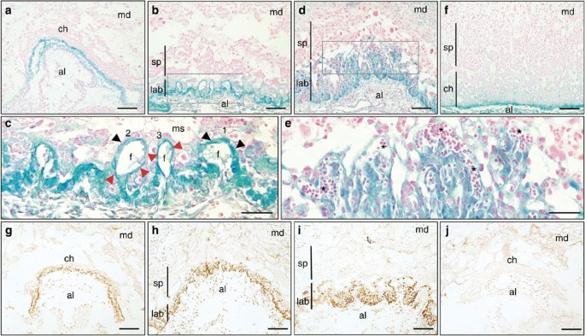Figure 5: Expression ofBcl9lis mainly restricted to ST-II and its precursor cells in the chorionic placenta. (a–j) β-Gal staining (a–f) or BCL9L immunostaining (g–j) of sections from E8.5 (a,g,j), E9.5 (b,h) and E10.5 (d,f,i) placentas. (a–e)Bcl9l+/−, (f,j)Bcl9l−/−and (g–i) wild-type. The boxed areas in panelsbanddare shown at higher magnification incande, respectively. Black arrowheads incindicate the layer of cells with an intermediate width of precursor cells and differentiated cells. Red arrowheads indicate elongated and thin ST-II. Numbers 1–3 incindicate the transition states of cells undergoing differentiation from precursor cells to ST-II. Asterisks ineindicate fetal red blood cells surrounded by β-gal-stained ST. al, allantois; ch, chorionic plate; f, fetal blood space; lab, labyrinth layer; md, maternal decidua; ms, maternal blood sinusoid; sp spongiotrophoblast. Scale bars, (c,e) 50 μm; (a,b,d,f–j) 100 μm. Figure 5: Expression of Bcl9l is mainly restricted to ST-II and its precursor cells in the chorionic placenta. ( a – j ) β-Gal staining ( a – f ) or BCL9L immunostaining ( g – j ) of sections from E8.5 ( a , g , j ), E9.5 ( b , h ) and E10.5 ( d , f , i ) placentas. ( a – e ) Bcl9l +/− , ( f , j ) Bcl9l −/− and ( g – i ) wild-type. The boxed areas in panels b and d are shown at higher magnification in c and e , respectively. Black arrowheads in c indicate the layer of cells with an intermediate width of precursor cells and differentiated cells. Red arrowheads indicate elongated and thin ST-II. Numbers 1–3 in c indicate the transition states of cells undergoing differentiation from precursor cells to ST-II. Asterisks in e indicate fetal red blood cells surrounded by β-gal-stained ST. al, allantois; ch, chorionic plate; f, fetal blood space; lab, labyrinth layer; md, maternal decidua; ms, maternal blood sinusoid; sp spongiotrophoblast. Scale bars, ( c , e ) 50 μm; ( a , b , d , f – j ) 100 μm. Full size image We also performed immunostaining using an antibody against BCL9L and found essentially the same cell type- and/or layer-specific expression pattern as seen by β-gal staining ( Fig. 5g–i ). Immunostaining revealed nuclear localization of BCL9L, and this staining was completely absent in the Bcl9l −/− sections ( Fig. 5j ). Consistent with the results from histological analyses, expression of BCL9L was completely absent in the spongiotrophoblast and the trophoblast giant cells as assessed by either β-gal staining or by BCL9L immunostaining. Thus, the expression pattern of BCL9L in the chorion basically coincides with those of Gcm1 and Synb [32] , [33] , consistent with the idea that BCL9L is an upstream regulator of the GCM1/syncytin pathway. Furthermore, strong and specific expression pattern of BCL9L in ST-II precursor and ST-II cells at E8.5 to 9.5 underscores the role of BCL9L in ST-II differentiation. The cell fusion pathway is dysregulated in Bcl9l −/− mice We next analysed the expression levels of Gcm1 and Synb as well as several trophoblast-specific marker genes in Bcl9l −/− placenta by qRT–PCR. Consistent with the marked proliferation and differentiation of trophoblast cells from E8.5 to 9.5, the expression levels of the genes examined increased accordingly ( Fig. 6a ). Throughout the stages examined, we observed striking decreases in Gcm1 and Synb expression (ca. 90% or more) in Bcl9l −/− placentas ( Fig. 6a ). By contrast, the expression of Syna , Dlx3 , Nr6a1 , Tpbp and Pl-1 was not affected ( Fig. 6a ). Although Dlx3 and Nr6a1 are broadly expressed among cell types in the labyrinth layer, Syna , Tpbp and Pl-1 are markers specific for ST-I and its precursor cells [33] , spongiotrophoblast, and trophoblast giant cells, respectively. These results further support the notion that BCL9L positively regulates the Gcm1/Synb pathway. 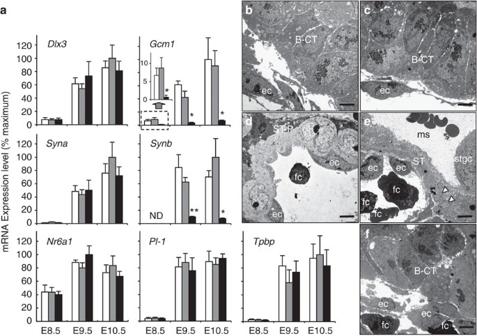Figure 6: Downregulation of the GCM1/syncytin-B pathway, and failure of fusion in the placenta ofBcl9l-deficient mice. (a) qRT–PCR analysis of trophoblast marker gene expression in the placentas of 4–6 concepti at different embryonic stages. Bars representingGcm1expression levels at E8.5 (dotted box) are magnified and shown above. ND, not detectable.SynBwere not detectable in approximately half of the samples of wild-type andBcl9l+/−and all ofBcl9l−/−at E8.5. Values were normalized byGAPDHexpression level and indicated as mean±s.e.m. *P<0.05; **P<0.005 (wild-type versusBcl9l−/−). Statistical tests were performed using the two-tailed Welch'st-test. Results without any indication are not statistically significant. Open bars represent wild-type, grey bars,Bcl9l+/−and black bars representBcl9l−/−. (b–f) Electron microscopic analysis of chorionic trophoblasts from E8.5 (b,c), E9.5 (d) and E10.5 (e,f) placentas. (b,f)Bcl9l−/−. (c–e)Bcl9l+/−. Note elongation and fusion of chorionic trophoblast cells inBcl9l+/−placenta at E9.5 (d), whereas basal chorionic trophoblast cells remain unfused and undifferentiated inBcl9l−/−placenta at E10.5 (f). Open arrowheads, nuclei of ST-II; B-CT, basal chorionic trophoblast; ec, fetal capillary endothelial cell; fc; fetal red blood cell; ms, maternal blood sinusoid; stgc, sinusoidal trophoblast giant cell; ST-P, ST precursor cells. Scale bars, (b–f) 5 μm. Figure 6: Downregulation of the GCM1/syncytin-B pathway, and failure of fusion in the placenta of Bcl9l -deficient mice. ( a ) qRT–PCR analysis of trophoblast marker gene expression in the placentas of 4–6 concepti at different embryonic stages. Bars representing Gcm1 expression levels at E8.5 (dotted box) are magnified and shown above. ND, not detectable. SynB were not detectable in approximately half of the samples of wild-type and Bcl9l +/− and all of Bcl9l −/− at E8.5. Values were normalized by GAPDH expression level and indicated as mean±s.e.m. * P <0.05; ** P <0.005 (wild-type versus Bcl9l −/− ). Statistical tests were performed using the two-tailed Welch's t -test. Results without any indication are not statistically significant. Open bars represent wild-type, grey bars, Bcl9l +/− and black bars represent Bcl9l −/− . ( b – f ) Electron microscopic analysis of chorionic trophoblasts from E8.5 ( b , c ), E9.5 ( d ) and E10.5 ( e , f ) placentas. ( b , f ) Bcl9l −/− . ( c – e ) Bcl9l +/− . Note elongation and fusion of chorionic trophoblast cells in Bcl9l +/− placenta at E9.5 ( d ), whereas basal chorionic trophoblast cells remain unfused and undifferentiated in Bcl9l −/− placenta at E10.5 ( f ). Open arrowheads, nuclei of ST-II; B-CT, basal chorionic trophoblast; ec, fetal capillary endothelial cell; fc; fetal red blood cell; ms, maternal blood sinusoid; stgc, sinusoidal trophoblast giant cell; ST-P, ST precursor cells. Scale bars, ( b – f ) 5 μm. Full size image The fusion of trophoblast cells into a multinucleated ST constitutes a critical step in the process of placental development [1] , [41] , [43] . We therefore examined fusion and morphological changes in trophoblast cells in Bcl9l −/− placentas by electron microscopy. At E8.5, chorionic trophoblasts from both Bcl9l −/− and control litters were observed to consist of polyhedral cell bodies, which were clearly separated from adjacent cells by plasma membranes and each of which contained a large nucleus ( Fig. 6b,c ). However, from E9.5 to 10.5, the basal chorionic trophoblast from Bcl9l −/− placentas did not undergo any major morphological changes or exhibit signs of differentiation, such as the appearance of numerous mitochondoria, large electron-dense globules or multi-nucleated syncytia [44] , as was observed in control litters ( Fig. 6d,e ; Supplementary Fig. S5 ). At E10.5, the chorionic trophoblast cells remained unfused and undifferentiated in Bcl9l −/− placentas ( Fig. 6f ). The placental phenotypes of Bcl9l -deficient mice were nearly identical to those reported for Gcm1 mutant mice [30] , [33] , which suggests that the mechanism underlying the placental defects in Bcl9l −/− concepti is due to the significant reduction in Gcm1 expression. As Gcm1 is an upstream regulator of Synb [33] , these results suggest that BCL9L regulates ST-II fusion and differentiation by positively regulating the GCM1/syncytin pathway. Furthermore, comparison of the phenotypes of mice mutant for various Wnt signalling components suggests that BCL9L may collaborate with frizzled5 [45] , a receptor for Wnt proteins, and R-spondin 3 (ref. 46 ), an activator of Wnt/β-catenin signalling. Notably, R-spondin 3 mutant mice also show a significant reduction in Gcm1 expression [46] . These similarities underscore the involvement of Wnt/β-catenin signalling in the regulation of Gcm1 expression and initiation of the branching morphogenesis in the placental labyrinth layer. In addition, as Pygo1/Pygo2 double-deficient mice have been reported not to show any major placental phenotype [47] , the role of BCL9L in placental morphogenesis is independent of the Pygo family of genes. This finding is consistent with previous reports showing that Pygo is dispensable for the transactivation activity of the BCL9 family of genes [23] , [48] . In some normal adult tissues, Wnt/β-catenin signalling activity has been shown to mainly reside in stem or progenitor cells and to increase upon injury [17] , [18] , [49] . Interestingly, stem or progenitor cells are suggested to be fusion partners of transplanted bone marrow-derived cells in tissue regeneration, at least in the intestine [3] . Moreover, in Min mice, which have a mutation of adenomatous polyposis coli that leads to constitutive activation of Wnt/β-catenin signalling, the frequency of fusion with bone marrow-derived cells in the intestine is increased compared with the wild-type [3] . We hypothesize that the β-catenin/GCM1/syncytin pathway-mediated cell fusion could be critical in some aspects of tissue regeneration and/or cancer development. Investigation of the involvement of the β-catenin/GCM1/syncytin pathway in tissue regeneration is underway in our laboratory. Plasmid constructs pTOP-tk-luciferase and pFOP-tk-luciferase were kind gifts from V Korinek and H Clevers. pRL-TK was from Promega, pMX-puro was a kind gift from T Kitamura and pBABE-puro (Addgene plasmid 1764, B. Weinberg) was from Addgene. pMX-β-catenin-S33Y and pMX-BCL9L were described elsewhere [23] . Human TCF4 cDNA was cloned into pBABE. luc-Int2-TBE10 was constructed by cloning the region containing TBE10 from intron 2 of the human GCM1 gene (52999306-53000227 of Genbank accession no. NC_000006.11) into Bam HI site of the pGL3-Promoter Vector (Promega). Site-directed mutation of TBE10 to produce luc-Int2-TBE10-mut was performed by using standard procedure. Antibodies Antibodies used were as follows: rabbit polyclonal antibody (pAb) to BCL9L (WB 1:2,000, IHC 1:3,000) was described elsewhere [23] ; briefly, polyclonal anti-BCL9L antibody was prepared by immunizing rabbits with a fragment of BCL9L (amino acids 245–564) fused to glutathione S -transferase. The antibody was purified with affinity chromatography using a column to which the antigen used for immunization had been linked. Rabbit polyclonal antibody to BCL9L is not available for distribution due to limited amount of stock. For other antibodies: mouse monoclonal antibody (mAb) to BCL9 (1:200, clone 2D4) was from Abnova; mouse mAb to β-catenin (1:1,000, clone 14) used in immunoblotting and mouse mAb to plakoglobin (1:500, clone 15) used in immunofluorescence were from BD Transduction Laboratories; goat pAb to TCF4 (1:1,500, N-20), rabbit pAb to Histone H3 (1:500, FL-136) and rabbit pAb to β-catenin (H102) used in ChIP assays were from Santa Cruz Biotechnology; mouse mAb to α-tubulin (1:500, clone DM1A) was from Calbiochem; rat mAb to CD31/PECAM (1:200, clone Mec13.3) was from BD Pharmingen; Alexa Fluor 594 Goat Anti-mouse IgG (1:500) and TO-PRO-3 (1:5,000) were from Molecular Probes. Cell culture and luciferase assays The human choriocarcinoma cell line BeWo was obtained from American Type Culture Collection and maintained as monolayers in 10 cm dish at 37 °C, 5% CO 2 with F-12K medium (Gibco) supplemented with 10% fetal bovine serum and 2 mM glutamine. Medium was changed daily to avoid depletion artifacts and 1/3 of the cells were passaged to new dishes every 3 days at subconfluency. For RNA interference experiments, 20–25 nM of siRNAs were reverse transfected into 6.5×10 4 BeWo cells per 500 μl in 24-well plates (or adjusted proportionally to the plate size) by Lipofectamine RNAiMAX (Invitrogen) according to the manufacturer's instructions. Untransfected samples are denoted as 'Mock' in the figures. At 24 and 48 h after transfection, medium was changed to that containing 50 μM FK or vehicle (dimethyl sulfoxide) and collected at 72 h post transfection for assay. Sequences for siRNA oligonuclotides are listed in Supplementary Table S2 . Stealth RNAi siRNA Negative Control Hi GC or Med GC was used as control siRNA. For TOP/FOP assays, transfections of plasmid constructs were performed using the Lipofectamine LTX (Invitrogen) according to the manufacturer's instructions at 48 h after reverse transfection of siRNAs. Briefly, 0.3 μg of pTOP- or pFOP-tk-luciferase was co-transfected with 0.1 μg of pRL-TK (internal control) using 0.5 μl of PLUS Reagent (Invitrogen) and 1.25 μl of LTX Reagent in a 48-well plate. For enhancer assays, 5.5×10 4 BeWo cells per 250 μl in 48-well plate were plated 24 h before transfection. Luc-Int2-TBE10 (0.15 μg) or luc-Int2-TBE10-mut (0.15 μg) and 0.05 μg of pRL-TK were co-transfected with the indicated expression vector or empty vector using 0.5 μl of PLUS Reagent and 1.25 μl of LTX Reagent. The symbol + in Figure 1h indicates transfection with 0.25 μg of plasmid DNA. Twenty-four hours after transfection of reporter plasmids, cells were collected and luciferase activities were measured using the Dual-Luciferase Reporter Assay System (Promega). Chromatin immunoprecipitation ChIP was performed according to Upstate Biotechnology's protocol (kit 17-925) with some modifications. Briefly, 1.8×10 6 BeWo cells per 10 ml were plated in 10 cm dish. When required, siRNA transfection was performed 72 h before the assays as described above. At 24 and 48 h after plating, medium was changed with that containing 50 μM FK or dimethyl sulfoxide. Cells were washed twice with ice-cold PBS containing proteinase inhibitors. Nuclear fractions were prepared as follows: Cells were suspended in 5× volume of cell lysis buffer (10 mM Hepes-KOH, pH 7.8, 10 mM KCl, 0.1 mM EDTA, 0.1% NP-40) and incubated for 5 min on ice. The suspension was centrifuged at 700 g for 3 min and then resuspended in 3× volume of cell lysis buffer using a 21-G syringe. The suspension was centrifuged at 700 g for 3 min and the nuclei sedimented were resuspended in 9.5 ml PBS. The nuclei were initially fixed by adding 0.5 ml of 20 mM DSP (dithiobis [succinimidyl propionate]; Pierce) and rotated for 30 min at 25 °C. The suspension was centrifuged at 190 g for 3 min and nuclei were fixed with 1% formaldehyde for 10 min at 25 °C. The reaction was stopped by adding 0.5 ml of 2.5 M glycine and rotating it for 5 min. The suspension was centrifuged at 700 g for 3 min and then resuspended in 0.3 ml nucleic lysis buffer (10 mM Tris–HCl, pH 7.5, 200 mM NaCl, 10 mM EDTA, 1% SDS) containing proteinase inhibitors. Lysates were sonicated to yield 300–1,000 bp DNA fragments. After elimination of cell debris by centrifugation, the sample was diluted with 1.8 ml of ChIP dilution buffer and was pre-cleared with 10 μl protein A-Sepharose (50% slurry) for 30 min at 4 °C with agitation. Precleared sample (0.1 ml) was saved to assess input DNA. Anti-β-catenin antibody (3 μg) was added to the precleared sample and gently mixed for 14 h at 4 °C, followed by rotation with 50 μl protein A-Sepharose slurry for 2 h. Subsequent wash, elution, protreinase K treatment and de-cross-linking procedures were performed according to the original protocol, except that de-cross-linking was performed for 14 h at 65 °C. ChIP-chip analysis SW480 was purchased from American Type Culture Collection and was cultured in RPMI 1640 medium containing 10% fetal bovine serum and 1% penicillin/streptomycin at 37 °C under 5% CO 2 . ChIP was performed as mentioned above. ChIP samples were amplified by in vitro transcription, labelled with biotin and hybridized to Human Tiling 2.0R Array A (Affymetrix) [50] , [51] . Briefly, ChIP DNA samples were amplified by two cycles of in vitro transcription using the T7 Megascript Kit (Ambion). The amplified RNA was converted into double-strand cDNA with random primers. Then cDNA was fragmented with DNase I and end-labelled with biotin. Input DNA (whole-cell extract) was prepared in the same manner. ChIP and input DNA samples were hybridized to arrays according to the manufacturer's instruction. After scanning and data extraction, enrichment values (ChIP/input DNA) were calculated using the model-based analysis of tiling-arrays algorithm [52] . The data are accessible through the GEO database under the accession number GSE29599. The list of putative target genes identified by ChIP-chip analysis is shown in Supplementary Data 1 . Cell fusion assay BeWo cells processed for siRNA procedures as mentioned above were fixed and immunostained by the standard procedure and were observed at a final magnification of ×400. Four (control) or eight (FK-treated) microscopic fields per sample were randomly selected for examination in each of three independent experiments. In general, a total of 200 (control) or 90 (FK-treated) nuclei were counted per field and, thus, nearly 700–800 nuclei were counted in each sample. A syncytium was defined as an agglomeration of two or more nuclei in the same cytoplasm without intervening plakoglobin membrane staining. Quantitative PCR For qRT–PCR, total RNA was extracted from mouse placentas or BeWo cells using Trisure reagent (Bioline). Reverse transcription was performed using the Superscript III (Invitrogen) or the ReverTra Ace (TOYOBO), respectively, by following the manufacturer's protocol. Real-time PCR was performed by using the LightCycler 480 Instrument (Roche) and LightCycler 480 SYBR Green I Master (Roche) according to the manufacturer's protocol. Primers used are listed in Supplementary Table S2 . Targeted disruption of the Bcl9l gene Genomic clones for the Bcl9l locus were isolated by screening of a C57BL/6N male liver genomic library (Clontech). The targeting vector was constructed by inserting a nuclear localization signal LacZ -polyA cassette followed by a loxP-flanked MC1 - neo -polyA cassette into 37-amino acids downstream of the first methionine, preserving 1.2 kb (5′) and 10.5 kb (3′) of the flanking region ( Supplementary Fig. S3 ). TT2 ES cells were electroporated and selected by standard procedure. Correctly targeted clones were screened by PCR, and subsequently confirmed by Southern blotting ( Supplementary Fig. S3 ). Targeted clones were used for aggregation with eight-cell embryos, and chimeric males were mated with C57BL/6N females. Subsequent genotyping was performed by genomic PCR ( Supplementary Fig. S3 ). Primers used are listed in Supplementary Table S2 . Heterozygotes were then backcrossed to C57BL/6N mice for at least nine generations. All animal experiments were conducted according to the Guidelines for care and use of animals, approved by the committee of The University of Tokyo. Immunostaining and microscopy Mouse concepti were dissected between E8.0 and E11.5 (day 0.5 was defined as noon of the day when the vaginal plug was detected) and placed in cold PBS. For histological analyses, placentas were fixed in 4% paraformaldehyde/PBS, embedded in paraffin and sectioned (8 μm), and then stained with haematoxylin and eosin. For immunohistochemical staining, placentas were fixed in 4% paraformaldehyde/PBS for 30–60 min, sequentially infiltrated with 10, 15 and 20% sucrose/PBS for >4 h each, then frozen in Tissue-Tek OCT compound (Sakura Finetek). Cryosections (10 μm) were used for antibody reaction and visualized using the Vectastain Elite ABC kit (Vector Laboratories) and diaminobenzidine. Sections from littermates were processed simultaneously on the same slide glass. For β-gal staining, placentas were fixed in 0.2% glutaraldehyde/PBS for 15 min, stained overnight at 37 °C in X-gal staining solution and subsequently counterstained with Nuclear Fast Red (Vector Laboratories). For electron microscopic analysis, placentas were prefixed with 2.5% glutaraldehyde/PBS (pH 7.2) for 3 h at 4 °C. Specimens were postfixed with 2% osmium tetroxide for 1 h and dehydrated in ethanol before being embedded in epoxy resin. Ultra-thin sections were stained with uranyl acetate and lead citrate and the grids were observed with a JOEL JEM1400 electron microscope operated at 100 kV. Statistical analysis Statistical analyses in this work were performed by an unpaired two-tailed Student's t -test or by a two-tailed Welch's t -test, where appropriate. A P -value of <0.05 was considered to be statistically significant. Acccession codes: The ChIP-chip data has been deposited in the GEO database under the accession code GSE29599 . How to cite this article: Matsuura K. et al . Identification of a link between Wnt/β-catenin signalling and the cell fusion pathway. Nat. Commun. 2:548 doi: 10.1038/ncomms1551 (2011).